Thymosin β4-sulfoxide attenuates inflammatory cell infiltration and promotes cardiac wound healing The downstream consequences of inflammation in the adult mammalian heart are formation of a non-functional scar, pathological remodelling and heart failure. In zebrafish, hydrogen peroxide released from a wound is the initial instructive chemotactic cue for the infiltration of inflammatory cells, however, the identity of a subsequent resolution signal(s), to attenuate chronic inflammation, remains unknown. Here we reveal that thymosin β4-sulfoxide lies downstream of hydrogen peroxide in the wounded fish and triggers depletion of inflammatory macrophages at the injury site. This function is conserved in the mouse and observed after cardiac injury, where it promotes wound healing and reduced scarring. In human T-cell/CD14+ monocyte co-cultures, thymosin β4-sulfoxide inhibits interferon-γ, and increases monocyte dispersal and cell death, likely by stimulating superoxide production. Thus, thymosin β4-sulfoxide is a putative target for therapeutic modulation of the immune response, resolution of fibrosis and cardiac repair. Cardiac injury activates an innate immune mechanism (reviewed in Frangogiannis [1] ) underpinned by sequential recruitment of inflammatory neutrophils and macrophages (leukocytes) to the site of injury. A direct consequence of immune cell infiltration is activation of fibroblasts and their differentiation to myofibroblasts, the principle source of collagen deposition, fibrosis and scarring. Recently, a study in the zebrafish revealed that the earliest ‘damage’ signal that instigates rapid neutrophil and macrophage influx to the wound is hydrogen peroxide (H 2 O 2 ) [2] . The identity of subsequent downstream signalling molecules or cues that encourage the resolution of immune cells away from the wound, once the acute phase is complete, remains unknown [3] . Thymosin β4 (Tβ4) is an actin-binding peptide, which exerts both anti-inflammatory and anti-fibrotic effects in the context of tissue wounding; notably following alkali eye injury [4] and blebomyocin-induced damage in the lung [5] . Tβ4 is one of the first proteins to be upregulated after wounding [6] and has been shown to modulate oxidative stress, targeting cardiac fibroblasts and cardiomyocyte survival following myocardial infarction [7] , [8] . There are two naturally occurring derivatives of Tβ4, the tetrapeptide Ac-SDKP, an N-terminal cleavage product known to have anti-fibrotic effects during hypertension [9] and which can reverse inflammation and fibrosis in rodents post MI [10] and Tβ4-sulfoxide (Tβ4-SO), formed by oxidation of the methionine-6 residue and thought to be the biologically active, secreted form of the parent peptide. Tβ4-SO is largely unstudied to-date, but has been shown to inhibit neutrophil chemotaxis in vitro and attenuate inflammation in carrageenan-injected mice [11] . We sought to investigate whether Tβ4-SO might act as the immune cell dispersal signal during cardiac wound healing to prevent chronic inflammation. Here we identify Tβ4-SO as downstream of H 2 O 2 acting to disperse inflammatory macrophages and promote healing following tail, body flank or heart injury in zebrafish. This function is conserved in mice, where Tβ4-SO, via a direct effect on leukocytes at key time points within healing myocardium, contributes to reduced fibrosis and scarring in the injured heart. Extrapolating these findings to humans, we show that Tβ4-SO blocks the production of pro-inflammatory IFN-γ to reduce the adhesion of activated monocytes and increases cell death downstream of elevated reactive oxygen species (ROS) production. Tβ4-SO acts downstream of H 2 O 2 in the wounded zebrafish We initially examined whether mechanical wounding of the zebrafish larval tail fin [2] would lead to production of Tβ4-SO in vivo . The zebrafish has five β-thymosin isoforms arising from successive rounds of gene duplication, [12] one of which has been described as the orthologue of Tβ4 ( Fig. 1a ), however, there are no previous reports describing Tβ4-SO in the zebrafish. Larvae at 72 h post fertilization (h.p.f.) were pre-incubated in the presence or absence of the small molecule inhibitor of H 2 O 2 diphenyleneiodium (DPI), followed by surgical removal of the tip of the tail fin ( Fig. 1b ). Levels of Tβ4-SO increased rapidly, 1 h post wounding, by approximately fivefold from 2% ± 1.4% s.e.m. to 10.4% ± 1.96% s.e.m. ( n =100 wounded tail fins per treatment, n =3 experimental replicates; Student’s t -test, P ≤0.01; Fig. 1c ). Pre-treatment with DPI resulted in a threefold increase (6.4% ± 0.8% s.e.m. ), which was significantly less than that observed in vehicle pre-treated control fish (Student’s t -test, P ≤0.05; Fig. 1d ). To investigate whether ectopic administration of Tβ4-SO might directly affect the presence of leukocytes, latex beads pre-adsorbed with synthetic Tβ4-SO or vehicle control (PBS), were implanted into Tg[mpo:GFP] zebrafish ( Fig. 1e ). Bead implantation acted as an injury stimulus resulting in recruitment of L-plastin+ (MPO−) macrophages [13] in the control setting ( Fig. 1g ). Imaging of fish at 3 and 6 h, thereafter, indicated a significantly reduced number of macrophages proximal to the Tβ4-SO bead relative to controls (3 h: co: 20±4.65 s.e.m. versus Tβ4-SO: 8.25±2.39 s.e.m. and 6 h: co:17.25±4.05 s.e.m. versus Tβ4-SO: 8.66±2.03 s.e.m. ( n =mean cell count from five bead-implanted fish per treatment; Student’s t -test, P ≤0.01; Fig. 1h ), suggesting ectopic Tβ4-SO either inhibited macrophage recruitment or acted to disperse macrophages at the implantation site. MPO+ neutrophil numbers were not significantly affected in this assay; normal neutrophil function involves stimulation of macrophage recruitment (reviewed in Soehnlein and Lindbom [14] ), suggesting Tβ4-SO was able to alter macrophage incidence despite the presence of neutrophils. 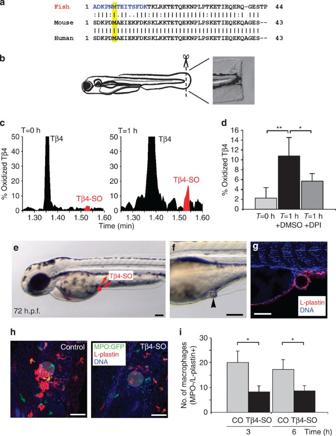Figure 1: Tβ4-SO acts downstream of H2O2and reduces macrophage accumulation in zebrafish wounds. Alignment of Tβ4 orthologues: highlighted in blue is the predicted trypsin-digest peptide fragment of the fish sequence for MS and in yellow the conserved methionine at position 6 (a). Schematic of the tail fin injury model at 72 h.p.f. and an example of a tail fin post wounding (b). Individual spectra from QTOF-MS of wounded tail fin samples, at time zero and 1 h post wounding, confirming detection and increase over time of parent Tβ4 and oxidized derivative Tβ4-SO (c). Quantification revealed a significant elevation in Tβ4-SO in wounded tissue after 1 h, which was abrogated by prior incubation with the H2O2inhibitor DPI (n=5 fishes per treatment, error bars are s.e.m. (d). Zebrafish larva at 72 h, indicating site of implantation of Tβ4-SO-soaked bead (e) and an actual bead in the lateral body wall (f). Bead implantation acted as a wound, as demonstrated by infiltration of L-plastin+ leukocytes (g). Immunostaining of fish 6 h post bead implantation revealed significant presence of neutrophils (MPO:GFP+), and macrophages (MPO−/L-plastin+) proximal to a control (vehicle-soaked) bead compared with a Tβ4-SO bead (h). Quantification of neutrophils and macrophages within a 500-μm radius of the bead wound site, revealed a significant reduction of MPO−/L-plastin+ macrophages proximal to Tβ4-SO beads as compared with controls at 3 and 6 h;n=5 fishes per treatment, error bars are s.e.m. (i). Scale bars, 100 μm (e); 100 μm (f); 150 μm (g); 20 μm (h). All statistics Student’st-test; *P≤0.05, **P≤0.01. Figure 1: Tβ4-SO acts downstream of H 2 O 2 and reduces macrophage accumulation in zebrafish wounds. Alignment of Tβ4 orthologues: highlighted in blue is the predicted trypsin-digest peptide fragment of the fish sequence for MS and in yellow the conserved methionine at position 6 ( a ). Schematic of the tail fin injury model at 72 h.p.f. and an example of a tail fin post wounding ( b ). Individual spectra from QTOF-MS of wounded tail fin samples, at time zero and 1 h post wounding, confirming detection and increase over time of parent Tβ4 and oxidized derivative Tβ4-SO ( c ). Quantification revealed a significant elevation in Tβ4-SO in wounded tissue after 1 h, which was abrogated by prior incubation with the H 2 O 2 inhibitor DPI ( n =5 fishes per treatment, error bars are s.e.m. ( d ). Zebrafish larva at 72 h, indicating site of implantation of Tβ4-SO-soaked bead ( e ) and an actual bead in the lateral body wall ( f ). Bead implantation acted as a wound, as demonstrated by infiltration of L-plastin+ leukocytes ( g ). Immunostaining of fish 6 h post bead implantation revealed significant presence of neutrophils (MPO:GFP+), and macrophages (MPO−/L-plastin+) proximal to a control (vehicle-soaked) bead compared with a Tβ4-SO bead ( h ). Quantification of neutrophils and macrophages within a 500-μm radius of the bead wound site, revealed a significant reduction of MPO−/L-plastin+ macrophages proximal to Tβ4-SO beads as compared with controls at 3 and 6 h; n =5 fishes per treatment, error bars are s.e.m. ( i ). Scale bars, 100 μm ( e ); 100 μm ( f ); 150 μm ( g ); 20 μm ( h ). All statistics Student’s t -test; * P ≤0.05, ** P ≤0.01. Full size image To address the issue of whether Tβ4-SO affected leukocyte recruitment versus dispersal, we generated time-lapse movies of the inflammatory cell response in Tg[LysC:dsRed] [15] larval zebrafish up to 4 h following bead implantation. While similar numbers of LysC+ leukocytes were recruited to the bead wound in the control and Tβ4-SO-treated setting at 1 and 2 h post injury, those that localized to a PBS bead were retained beyond 3 h post injury, whereas those that encountered a Tβ4-SO-coated bead dispersed at and beyond this time point, suggesting the latter did not inhibit the initial inflammatory cell recruitment but rather induced their subsequent resolution ( Supplementary Fig. S1 ; Supplementary Movies 1 and 2 ). Extrapolating from generic tissue wounding, we next examined the leukocyte response in a model of zebrafish heart injury. Both laser- and needle-induced injuries in the larval heart at 72 h resulted in the release of H 2 O 2 from the wound site, as determined by free radical spin trap analysis with 5,5-dimethyl-1-pyrroline- N -oxide (DMPO; Fig. 2a ). Delivery of Tβ4-SO or PBS control via microinjection or bathing of the larvae in Tβ4-SO-containing medium, resulted in significantly reduced incidence of infiltrating leukocytes (L-plastin+) at both 3 and 6 h post injury (3 h: co: 30.4±2.96 s.e.m. versus Tβ4-SO: 22.5±1.50 s.e.m. ; Student’s t -test, P ≤0.05 and 6 h: co: 35.3±3.19 s.e.m. versus Tβ4-SO: 18.2±1.90 s.e.m. ; Student’s t -test, P ≤0.01; n =mean cell count from four injured fish per treatment; Fig. 2b–f ). 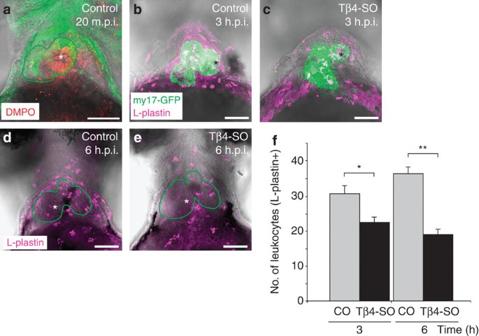Figure 2: Tβ4-SO disperses leukocytes after cardiac injury in zebrafish. (a) Laser injury to the heart of a 72-h zebrafish larvae immunostained for DMPO (red) revealed localized H2O2production at the wound site (b). At 3 h post laser heart injury (h.p.i.), a reduced leukocytic response (revealed by L-plastin staining – magenta;c,d) was seen in Tβ4-SO-treated fish within 500 μm of the focal point of injury (c) compared with controls (b). Larger, needle-induced wounds to the heart region ofTg[myl7:GFP]transgenic fish, resulted in a stronger inflammatory response in PBS-treated control hearts at 6 h.p.i. (d), which was significantly reduced in Tβ4-SO-treated fish (e). Total numbers of L-plastin+ leukocytes was significantly lower at 3 and 6 h.p.i. for Tβ4-SO-treated fish compared with controls;n=5 fishes per treatment, error bars are s.e.m. (f). Asterisks mark wound site and green outlines delineate the heart as determined by myl7-GFP+. Scale bars, 100 μm (a–e). All statistics Student’st-test; *P≤0.05, **P≤0.01. Figure 2: Tβ4-SO disperses leukocytes after cardiac injury in zebrafish. ( a ) Laser injury to the heart of a 72-h zebrafish larvae immunostained for DMPO (red) revealed localized H 2 O 2 production at the wound site ( b ). At 3 h post laser heart injury (h.p.i. ), a reduced leukocytic response (revealed by L-plastin staining – magenta; c , d ) was seen in Tβ4-SO-treated fish within 500 μm of the focal point of injury ( c ) compared with controls ( b ). Larger, needle-induced wounds to the heart region of Tg[myl7:GFP] transgenic fish, resulted in a stronger inflammatory response in PBS-treated control hearts at 6 h.p.i. ( d ), which was significantly reduced in Tβ4-SO-treated fish ( e ). Total numbers of L-plastin+ leukocytes was significantly lower at 3 and 6 h.p.i. for Tβ4-SO-treated fish compared with controls; n =5 fishes per treatment, error bars are s.e.m. ( f ). Asterisks mark wound site and green outlines delineate the heart as determined by myl7-GFP+. Scale bars, 100 μm ( a – e ). All statistics Student’s t -test; * P ≤0.05, ** P ≤0.01. Full size image Tβ4 and Tβ4-SO reduce inflammatory cell infiltration after MI To investigate the effect of Tβ4-SO on leukocyte infiltration during wounding in mammals, we utilized the mouse MI model. It is known that two distinct phases of monocytes participate post MI in the mouse: inflammatory monocytes (Ly-6C hi ) dominate during the early phase I (days 1–3) and exhibit phagocytic and proteolytic function to digest damaged tissue, whereas monocytes with attenuated inflammatory properties (Ly-6 lo ) dominate later (from days 4–7) during the wound-healing phase II [16] . Hence, we focused on these key time points and on the potential for the parent peptide Tβ4 and derivative Tβ4-SO to augment the transition from phase I to II. We initially treated animals with Tβ4 immediately post MI and compared against both vehicle-treated controls and Tβ4 global knockout (equivalent to loss of Tβ4-SO function) mice. MPO+ neutrophils increased in the border zone of the infarct by day 2 and peaked at day 4 post injury for all mice. Tβ4 treatment attenuated this increase with fewer MPO+ cells present (co: 70±14.5 s.e.m. versus Tβ4: 30±19.1 s.e.m., P ≤0.15) at the site of injury at both stages ( Fig. 3a–d ). Global knockout of Tβ4 significantly increased MPO+ cell numbers at the earliest stages of infiltration (day 2; wild type: 20.5±4.6 s.e.m. versus Tβ4 KO: 47.7±5.0 s.e.m. ; Student’s t -test, P ≤0.01), thereafter, numbers were equivalent to that observed for control (vehicle-treated) mice ( Fig. 3a–d ). We next investigated the levels of TNF-α, as the upstream cytokine responsible for initiating the inflammatory cascade [17] . TNF-α was significantly reduced (6.2-fold reduction) after 2 days of Tβ4 treatment post MI as compared with vehicle controls ( Fig. 3e ), as was the downstream pro-inflammatory cytokine IL-6 (4.1-fold reduction), which ordinarily is rapidly induced in the ischaemic myocardium ( Fig. 3e ). In keeping with the role in mitigating inflammatory injury during the early stages post infarct, without interfering with subsequent myocardial healing, Tβ4 stimulated the expression of the inhibitory cytokine IL-10 at 2 days post MI (8.1-fold increase compared with control; Fig. 3e ). In control mice, the number of F4/80+ macrophages significantly increased between days 2–7 post MI ( Fig. 3g ). Treatment with Tβ4 resulted in an initial increase in F4/80+ cells at day 2 ( Fig. 3i ), peaking at day 4 post MI, followed by a significant reduction at day 7 post MI (co: 21±3.4 s.e.m. versus Tβ4: 3±1.4 s.e.m. ; Student’s t -test, P ≤0.05; Fig. 3m ). In Tβ4 knockout mice, we observed the opposite effect, such that F4/80+ cells increased continuously to around fivefold that of control mice by day 7 post MI (21±3.4 s.e.m. versus 135.8±12.4 s.e.m. ; Student’s t -test, P ≤0.001; Fig. 3k ). The observation that Tβ4 efficiently cleared the macrophage-rich infiltrate by day 7 post MI was consistent with the zebrafish data for Tβ4-SO ( Fig. 1h ). 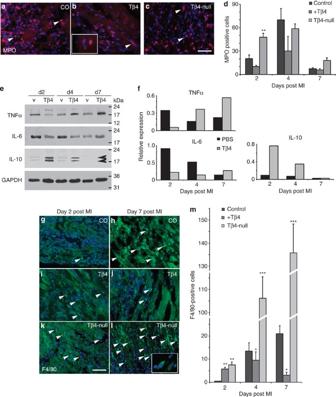Figure 3: Tβ4/Tβ4-SO modulates the inflammatory response post MI in the mouse heart. Representative images, showing infiltration of the injured myocardium with neutrophils (white arrowheads highlight individual MPO+ cells;a–c) and macrophages (white arrowheads highlight individual F4/80 cells;g–l) in Tβ4-treated, control vehicle-treated and Tβ4-null myocardial infarction (MI) hearts. Significantly fewer cytotoxic myeloperoxidase (MPO)-peroxidase+ neutrophils were present in Tβ4-treated, compared with controls and Tβ4-null hearts at days 2 and 4 post MI (a–d). Inset inbillustrates specific MPO staining of a neutrophil at higher magnification. Significantly more neutrophils were present at the infarct site in the Tβ4-null hearts at day 2, consistent with the timing of initial inflammatory cell infiltration (d). Western blots for TNF-α, IL-6, IL-10 and GAPDH at 2, 4 and 7 days post MI in animals treated with Tβ4 as compared with vehicle controls (e) and quantification of protein expression by scanning densitometry (f). Black arrowheads indicate alternate glycosylated isoforms (21 and 24 kDa) of IL-10. The upstream initiator of the acute inflammatory cascade, TNF-α, is downregulated at early stages post MI (2 days) following Tβ4 treatment along with the downstream inflammatory cytokine, IL-6; levels of both TNFα and IL-6 subsequently become elevated after 7 days consistent with an early reduction in injury and enhanced repair at later stages (e,f). The anti-inflammatory cytokine IL-10 is upregulated after 2 and 4 days of treatment with Tβ4 (e,f). Representative images, F4/80-positive macrophages in the scar region post MI, in co (g,h), Tβ4-treated (i,j) or Tβ4−/−animals (k,l); both at day 2 (g,i,k) and day 7 (h,j,l) post MI, with cell counts quantified inm. Tβ4-induced macrophage infiltration peaks at day 4 but is rapidly cleared, to a level significantly reduced relative to vehicle treated by day 7; in Tβ4-null hearts the incidence of macrophages at the wound was significantly elevated relative to the controls as highlighted by cell counts (m). Scale bar, 20 μm (a–c) and 20 μm (g–l); v, vehicle.n=4–6 MI hearts analysed per time point; error bars are s.e.m. for all bar graphs; all statistics Student’st-test; *P≤0.05, **P≤0.01, ***P≤0.001. Figure 3: Tβ4/Tβ4-SO modulates the inflammatory response post MI in the mouse heart. Representative images, showing infiltration of the injured myocardium with neutrophils (white arrowheads highlight individual MPO+ cells; a – c ) and macrophages (white arrowheads highlight individual F4/80 cells; g – l ) in Tβ4-treated, control vehicle-treated and Tβ4-null myocardial infarction (MI) hearts. Significantly fewer cytotoxic myeloperoxidase (MPO)-peroxidase+ neutrophils were present in Tβ4-treated, compared with controls and Tβ4-null hearts at days 2 and 4 post MI ( a – d ). Inset in b illustrates specific MPO staining of a neutrophil at higher magnification. Significantly more neutrophils were present at the infarct site in the Tβ4-null hearts at day 2, consistent with the timing of initial inflammatory cell infiltration ( d ). Western blots for TNF-α, IL-6, IL-10 and GAPDH at 2, 4 and 7 days post MI in animals treated with Tβ4 as compared with vehicle controls ( e ) and quantification of protein expression by scanning densitometry ( f ). Black arrowheads indicate alternate glycosylated isoforms (21 and 24 kDa) of IL-10. The upstream initiator of the acute inflammatory cascade, TNF-α, is downregulated at early stages post MI (2 days) following Tβ4 treatment along with the downstream inflammatory cytokine, IL-6; levels of both TNFα and IL-6 subsequently become elevated after 7 days consistent with an early reduction in injury and enhanced repair at later stages ( e , f ). The anti-inflammatory cytokine IL-10 is upregulated after 2 and 4 days of treatment with Tβ4 ( e , f ). Representative images, F4/80-positive macrophages in the scar region post MI, in co ( g , h ), Tβ4-treated ( i , j ) or Tβ4 −/− animals ( k , l ); both at day 2 ( g , i , k ) and day 7 ( h , j , l ) post MI, with cell counts quantified in m . Tβ4-induced macrophage infiltration peaks at day 4 but is rapidly cleared, to a level significantly reduced relative to vehicle treated by day 7; in Tβ4-null hearts the incidence of macrophages at the wound was significantly elevated relative to the controls as highlighted by cell counts ( m ). Scale bar, 20 μm ( a – c ) and 20 μm ( g – l ); v, vehicle. n =4–6 MI hearts analysed per time point; error bars are s.e.m. for all bar graphs; all statistics Student’s t -test; * P ≤0.05, ** P ≤0.01, *** P ≤0.001. Full size image We next investigated the anti-inflammatory activity of Tβ4-SO by flow cytometry of infarct cell suspensions and observed an early (day 2) significant increase in F4/80+ cells (co: 23.0%±2.85% s.e.m. versus Tβ4-SO: 32.0%±2% s.e.m. ; n =4; Student’s t -test, P ≤0.05; Fig. 4a ), which represented an increase in the proportion of macrophages, as the total number of monocyte (CD11b hi , (Ly6G, B220, CD49b, CD90.2, NK1.1) low ) cells remained unaltered ( Fig. 4b ). Conversely, 4 days post injury the total number of monocytes was significantly reduced compared with controls (co: 5.9%±0.95% s.e.m. versus Tβ4-SO: 2.7%±0.4% s.e.m. ; n =4; Student’s t -test, P ≤0.05; Fig. 4c ). Tβ4-SO treatment of infarct suspensions did not, however, alter the relative proportions of monocyte Ly-6 lo versus Ly-6C hi sub-populations within the reduced infiltrate at days 2 and 4 post MI ( Supplementary Fig. S2a,b ). 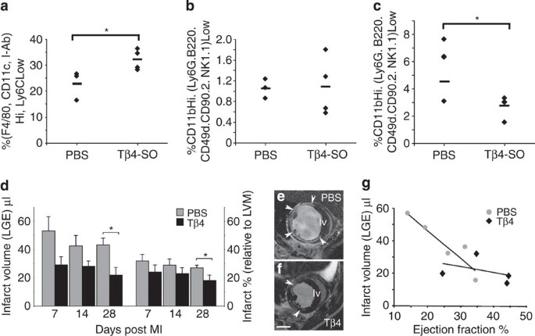Figure 4: Tβ4/Tβ4-SO attenuates inflammatory cell infiltration, scarring and fibrosis. Following treatment with Tβ4-SO, FACS analyses at 2 days post MI revealed a significant increase in macrophages at day 2 post MI (a), with no change in the total number of monocytes recruited (b). In MI samples, 4 days post injury the total number of monocytes was significantly reduced (c). Tβ4 treatment resulted in significantly increased Tβ4-SO levels (refer to main text) and reduced scarring and fibrosis, by 28 days post MI, according to surrogate measures of infarct volume and % infarct relative to LVM (LVM); as determined by longitudinal MRI of LGE;n=4 hearts per treatment per time point; error bars are s.e.m. (d). Short-axis MRI images of PBS control (e) and Tβ4 (f) treated hearts at day 28 post MI highlighted the extent of infarct and fibrosis (white arrowheads) in the wall of the left ventricle (lv), which is reduced in Tβ4-treated animals (comparingewithf). Infarct volume negatively correlated with ejection fraction at day 28 MI, consistent with the late remodelling phase and reduced LGE in Tβ4-treated hearts (slope: −0.37;P=0.624) compared with PBS controls (slope: −1.76;P=0.0234) reflected reduced scar formation (g). Scale bar, 2 mm (f). Statistics repeated measures one-way analysis of variance; *P≤0.05. Figure 4: Tβ4/Tβ4-SO attenuates inflammatory cell infiltration, scarring and fibrosis. Following treatment with Tβ4-SO, FACS analyses at 2 days post MI revealed a significant increase in macrophages at day 2 post MI ( a ), with no change in the total number of monocytes recruited ( b ). In MI samples, 4 days post injury the total number of monocytes was significantly reduced ( c ). Tβ4 treatment resulted in significantly increased Tβ4-SO levels (refer to main text) and reduced scarring and fibrosis, by 28 days post MI, according to surrogate measures of infarct volume and % infarct relative to LVM (LVM); as determined by longitudinal MRI of LGE; n =4 hearts per treatment per time point; error bars are s.e.m. ( d ). Short-axis MRI images of PBS control ( e ) and Tβ4 ( f ) treated hearts at day 28 post MI highlighted the extent of infarct and fibrosis (white arrowheads) in the wall of the left ventricle (lv), which is reduced in Tβ4-treated animals (comparing e with f ). Infarct volume negatively correlated with ejection fraction at day 28 MI, consistent with the late remodelling phase and reduced LGE in Tβ4-treated hearts (slope: −0.37; P =0.624) compared with PBS controls (slope: −1.76; P =0.0234) reflected reduced scar formation ( g ). Scale bar, 2 mm ( f ). Statistics repeated measures one-way analysis of variance; * P ≤0.05. Full size image These data are consistent with a bi-phasic effect of the influence of Tβ4/Tβ4-SO. During the so-called debris-removal phase 1 (day 2), Tβ4/Tβ4-SO increased macrophage numbers by directing transformation of the stable monocyte pool and subsequently enhanced the transition to the anti-inflammatory phase II (day 4) by signalling monocyte/macrophage clearance from the injury site. A Tβ4/Tβ4-SO-depleted monocyte infiltrate reduces scarring The functional consequences of the Tβ4/Tβ4-SO-depleted monocyte infiltrate were examined by serial MRI of mice treated with Tβ4, to reflect sulfoxide activity, for 7, 14 and 28 days post MI. Tβ4-SO was increased in hearts following the addition of Tβ4 across the time course of the study: percentage oxidized Tβ4 increased from 4.7±1.3% in sham control hearts to 66±5.1% at day 2 post MI, maintained at an equivalent elevated level (68.6±9.3%) through to 28 days post MI ( n =4; repeated measures one-way analysis of variance; P ≤0.001). Increase in infarct volume (late gadolinium enhancement; LGE) was significantly higher in PBS compared with Tβ4-treated mice; persisting up to day 28 post MI (co: 43.3±4.9 μl; n =5 versus Tβ4: 22.0±5.3 μl; n =4; Student’s t -test; P ≤0.05; Fig. 4d ) and % infarct relative to left ventricular mass (LVM) followed the same trend (day 28 post MI: co: 27±2%; n =5 versus Tβ4: 18±4%; n =4; Student’s t -test, P ≤0.05; Fig. 4d ) indicating that Tβ4/Tβ4-SO reduced infarct size and scarring. The reduced fibrosis was confirmed in the free ventricular wall following Tβ4 treatment ( Fig. 4e ), which, in turn, directly correlated with improved cardiac function as indicated by elevated ejection fraction ( Fig. 4g ). Tβ4-SO has anti-inflammatory effects on human monocytes Extrapolating the animal model findings to human monocytes/macrophages, we investigated the response to inflammatory stimuli in the presence of Tβ4-SO. Interactions between CD4+ T cells and monocyte/macrophages are known to drive pro-inflammatory and anti-inflammatory responses [18] . We established co-cultures of CD4+ T cells and CD14+ monocytes from the peripheral blood mononuclear cells of healthy individuals and initially excluded any effect of Tβ4 or Tβ4-SO on the underlying T cells ( Supplementary Fig. S3 ) or the monocyte inflammatory phenotype per se via activation or differentiation ( Supplementary Fig. S4 ). The addition of Tβ4-SO lead to a significant reduction in the release of the pro-inflammatory cytokine IFN-γ, relative to controls (co: 1,830 pg ml −1 ± 365.3 pg ml −1 s.e.m. versus Tβ4-SO: 1,271.5 pg ml −1 ± 483.1 s.e.m., n =4; Wilcoxon matched-pairs signed rank test, P ≤0.05; Fig. 5a ). IFN-γ is secreted by T cells and functions to both activate macrophages and establish conditions of adhesion and binding required for their migration (reviewed in Schroder et al . [19] ). CD14+ cells treated with Tβ4-SO were significantly less adherent than their control counterparts, even in the presence of recombinant IFN-γ (co: 219,167±25,834 s.e.m. versus Tβ4-SO: 89,167±13,411 s.e.m. ; n =3; Student’s t -test, P ≤0.05; Fig. 5b ). We next assessed whether effects on CD14+ cell adhesion/dispersal might be accompanied by elevated cell death and observed Tβ4-SO significantly increased the number of trypan blue-positive cells compared with IFN-γ and control treated cultures (Tβ4-SO: 135,833±22,928 s.e.m. versus IFN-γ: 55,833±2,203 s.e.m. versus co: 33,333 ± 833 s.e.m. ; n =3; P ≤0.05; Fig. 5d ). To determine a potential mechanism, we investigated whether Tβ4-SO, in the presence of IFN-γ, might act to increase intracellular ROS and thus provoke oxidative stress-induced apoptosis [20] . Increased ROS is known to occur downstream of H 2 O 2 release and cell survival can be maintained by reversal of H 2 O 2 -induced oxidation of methionine [21] . Macrophages from the peritoneal cavity of mice were stimulated with IFN-γ and incubated with either vehicle or Tβ4-SO followed by dihydroethidium, a fluorescent indicator of ROS [22] . Activating IFN-γ treatment alone resulted in increased ROS, which was significantly augmented by the addition of Tβ4-SO ( n =3; Student’s t -test, P ≤0.05; Fig. 5e ); consistent with Tβ4-SO acting downstream of H 2 O 2 -methionine oxidation and oxidative stress. 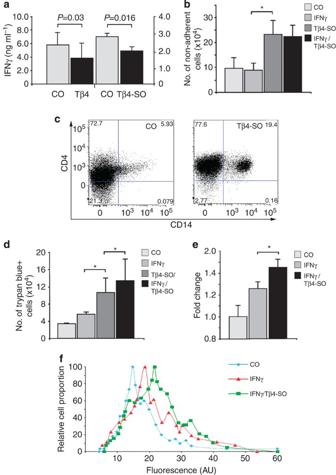Figure 5: Tβ4-SO reduces adhesion and increases cell death of human monocytes via increased ROS. Co-cultures of human CD14+ monocytes and CD4+ T cells treated with either Tβ4 or Tβ4-SO resulted in significantly decreased levels of IFNγ;n=4 co-cultures per treatment; error bars are s.e.m. (a). In both single CD14+ monocyte cultures and co-cultures with CD4+ T cells, Tβ4-SO significantly reduced the adherence of the cells in the presence of IFNγ;n=3 cultures per treatment; error bars are s.e.m. (b,c); presence of cells in the right FACS quadrant reflects non-adherent monocytes when treated with Tβ4-SO (c). Vital dye staining (trypan blue) of CD14+ cultures demonstrated Tβ4-SO significantly increased monocyte cell death, which was further increased by the additive effect of IFNγ;n=3 cultures per treatment; error bars are s.e.m. (d). In isolated murine peritoneal macrophages, Tβ4-SO resulted in a significant fold increase in ROS;n=3 cultures per treatment; error bars are s.e.m. (e), which was reflected by increased dihydroethidium fluorescence (f). Statistics: Wilcoxon matched-pairs signed rank test (a) and Student’st-test (b,d,e); *P≤0.05. Figure 5: Tβ4-SO reduces adhesion and increases cell death of human monocytes via increased ROS. Co-cultures of human CD14+ monocytes and CD4+ T cells treated with either Tβ4 or Tβ4-SO resulted in significantly decreased levels of IFNγ; n =4 co-cultures per treatment; error bars are s.e.m. ( a ). In both single CD14+ monocyte cultures and co-cultures with CD4+ T cells, Tβ4-SO significantly reduced the adherence of the cells in the presence of IFNγ; n =3 cultures per treatment; error bars are s.e.m. ( b , c ); presence of cells in the right FACS quadrant reflects non-adherent monocytes when treated with Tβ4-SO ( c ). Vital dye staining (trypan blue) of CD14+ cultures demonstrated Tβ4-SO significantly increased monocyte cell death, which was further increased by the additive effect of IFNγ; n =3 cultures per treatment; error bars are s.e.m. ( d ). In isolated murine peritoneal macrophages, Tβ4-SO resulted in a significant fold increase in ROS; n =3 cultures per treatment; error bars are s.e.m. ( e ), which was reflected by increased dihydroethidium fluorescence ( f ). Statistics: Wilcoxon matched-pairs signed rank test ( a ) and Student’s t -test ( b , d , e ); * P ≤0.05. Full size image Despite a number of previous studies assigning anti-inflammatory and anti-fibrotic properties to Tβ4, there remains no insight as to how this peptide might mediate effects directly on the innate immune-cell response post wounding. Here we sought to test the hypothesis that a naturally occurring oxidized derivative, Tβ4-SO, might act to disperse inflammatory cells from sites of injury in a conserved manner from zebrafish, through rodents, to man. This study was underpinned by prior identification of H 2 O 2 as the initial chemo-attractive signal for recruitment of inflammatory cells to a wound [2] and the outstanding question as to what might be the downstream factor responsible for resolving these cells to prevent chronic inflammation [3] . Tβ4-SO is formed by methionine oxidation of Tβ4 in the presence of H 2 O 2 , which alongside the observed upregulation of Tβ4 at wound sites [6] , [23] established the sulfoxide variant as a potential candidate for immune cell dispersal. We initially generated a simple zebrafish tail fin resection model [2] and revealed by QTOF-MS that Tβ4-SO is significantly upregulated post wounding in zebrafish in a H 2 O 2 -dependent manner. In subsequent zebrafish lateral body wall and heart injury models, ectopic sulfoxide induced the resolution of leukocytes/macrophages from the site of injury downstream of H 2 O 2 . Thus, Tβ4-SO may function as the elusive dispersal signal to prevent chronic inflammation and promote wound healing. Extrapolating to mouse MI, both the parent molecule Tβ4 and sulfoxide derivative were necessary and sufficient to ensure an elevated presence of macrophages, within the stable (Ly-6C hi ) monocyte pool, during the debris and necrotic tissue-removal phase I, followed by significantly increased clearance during the transition to the wound-healing phase II following cardiac injury [16] . These findings collectively suggest Tβ4 through conversion to Tβ4-SO can function to prevent monocytosis and, therefore, excessive granulation tissue formation as an immediate downstream consequence [16] . Functionally, the altered inflammatory infiltrate likely contributes to the reduced fibrosis and scarring, as determined by MRI, and as previously described [16] . However, Tβ4 is also known to promote a range of reparative functions post MI, which will have a significant impact here; including the maintenance of cardiomyocyte survival via Akt signalling [24] , the induction of neo-vascularisation and coronary angiogenesis [25] , [26] and reactivation of adult epicardial cells to contribute to myocardial regeneration [27] . Thus, the anti-inflammatory role described for Tβ4-SO is one of a number of contributory factors reflecting the pleiotropy of Tβ4 in the context of cardiac wound healing and repair. Mechanistically, we observed no effect of either Tβ4/Tβ4-SO on monocyte activation or differentiation, as determined by flow sorting against a signature set of markers (CD16, CD40, HLA-DR, CD54, CD86, CD163, CD206). In human co-cultures the clearance and dispersal was dependent upon a combination of modulating IFN-γ-induced cell adhesion, favouring increased human CD14+ monocyte migration, and cell death supported by increased vital dye staining and elevated ROS-mediated apoptosis in murine splenic monocytes. Inflammatory cells are in fact known to release ROS to kill locally invading microbes to prevent infection of wounds [28] ; here we introduce the concept of co-opting ROS killing to feedback onto the resolution of the immune cells themselves. In summary, post-infarction immune cells are required for the transition into a reparative phase, however, their persistence can lead to chronic inflammation, characterized by excessive granulation tissue/scar, attenuated repair and long-term pathological remodelling of the injured heart (reviewed in Frangogiannis et al . [29] and Aoki et al . [30] ). Consequently, timely resolution of the inflammatory infiltrate is essential for optimal infarct healing. Our data are consistent with the Tβ4-SO, formed as a by-product of H 2 O 2 production from the wound site, acting to resolve immune cells and modulate cardiac fibrosis and scarring. MS analysis of Tβ4-SO At 72 h.p.f., zebrafish were pre-treated for 30 min with either 10 μM DPI or DMSO followed by resection of the caudal fin. The fish were recovered for 1 h followed by removal of a small section of tissue immediately proximal to the wound. The tissue was reconstituted in 20 μl of 100 mM Tris, pH 7.8, containing 8 M urea, vortexed for 1 h, and 1.5 μl of 0.2 M dithioerythritol in 100 mM Tris, pH 7.8 was added, vortexed again and the sample incubated at room temperature for 1 h. A volume of 3 μl of 0.2 M iodoacetamide in 100 mM Tris, pH 7.8 was added, vortexed and incubated for 30 min at room temperature. Finally, 165 μl of H 2 O containing 1 μg of proteomics grade trypsin (Sigma) was added and incubated for ≥16 h at 37 °C. Separation of samples and standards was performed using a 2795XE high-performance liquid chromatography (HPLC; Waters, UK). The HPLC protocol: isocratic gradient of 95% dH 2 O: 5% acetonitrile over a 55-min period; flow rate 0.5 ml min −1 , diverted to waste for the first 1.5 min after sample injection, to minimize accumulation of endogenous compounds on the ionization source. The HPLC was coupled to a triple quadrupole tandem mass spectrometer (MicroMass Quattro; Waters) operating in negative-ion mode using the following settings: capillary 3.2 kV, source temperature 150 °C, desolvation temperature 350 °C, cone voltage 30 V, cone gas flow rate 90 l h −1 and desolvation gas flow rate 900 l h −1 . The MRM mode was used for quantification and data were acquired and processed using MassLynx software (Waters). In vivo analysis of leukocyte recruitment in zebrafish Zebrafish were housed and maintained in environmentally controlled aquaria. All surgical and pharmacological procedures were performed in accordance with the Animals (Scientific Procedures) Act 1986 (A(SP)A; Home Office, UK). Wild-type, Tg(mpo:GFP), Tg[LysC:dsRed] or Tg(myl7:GFP) zebrafish larvae (72 h.p.f.) were anesthetized in MS-222 and placed in 3% methyl cellulose in 0.3% Danieau’s solution on a glass slide. Heparin-Ceramic HyperD M Hydrogel Composite beads (Sigma-Aldrich, H0532) were rinsed for 5–10 min in 0.3% Danieau’s solution five times and pre-soaked in 100 μg ml −1 Tβ4-SO or PBS for 30 min+ before being inserted through the skin and muscle of the flank region using a fine tungsten needle (World Precision Instruments). Heart injury was either via microinjection delivery of Tβ4-SO (3 nl of 100 μg ml −1 ) into the heart and pericardial space or implanting of a bead into this region, as described above. Control fish were injected with PBS vehicle or beads soaked in PBS vehicle. For laser injury, fish were pre-treated with 100 μg ml −1 of Tβ4-SO or PBS in Danieau’s solution for at least 2 h, embedded in low-gelling point Agarose (Sigma-Aldrich, A9414) and wounded using a nitrogen ablation laser (Spectra-Physics) attached to a Zeiss Axioplan 2 wide-field imaging system. For imaging of H 2 O 2 production, 72 h.p.f. Tg(myl7:GFP) larvae were incubated in Danieau’s medium containing 200 mM DMPO (Enzo Life Sciences) for 5 h, wounded and then killed at 30 m.p.i. Larvae were fixed in 4% paraformaldehyde overnight at 4 °C and subjected to whole-mount immunostaining using rabbit anti-L-plastin (1:500), rabbit anti-DMPO (1:200; ALX-210-530-R050, Enzo Life Sciences) or chicken anti-GFP antibodies (1:200; Invitrogen, A10262). Secondary antibodies: Alexa Fluor 546 or 647 goat anti-rabbit and Alexa Fluor 647 goat anti-chicken (all 1:200; Invitrogen, A11035, A21245, A21449, respectively). Images were taken using a Leica SP5 confocal imaging system attached to a Leica DMI 6000 inverted microscope. For live imaging of LysC:dsRED+ positive leukocyte recruitment to a wound, fish were anesthetized and a bead inserted as described above. Fish were then embedded in low-gelling point agarose and imaged using the Leica confocal system. Immune cell numbers within a 500-μm radius of the wound site were counted manually using Fiji software. Myocardial infarction Mice were housed and maintained in a controlled environment. All surgical and pharmacological procedures were performed in accordance with the Animals (Scientific Procedures) Act 1986 (A(SP)A; Home Office, UK). Myocardial infarction was induced in isoflurane-anaesthetized mice by permanent ligation of the left anterior descending artery. On recovery, animals received interperitoneal (i.p.) injection of either Tβ4 (6 mg kg −1 ), Tβ4-SO (6 mg kg −1 ) or vehicle (PBS). Further injections were given every second day unless otherwise stated. Hearts were harvested at 2, 4 and 7 days after ligation and either prepared for flow cytometry or immunofluorescence. Immunofluorescent quantification of cells in MI hearts Immunofluorescence was performed on hearts post MI. Hearts were first fixed in 4% paraformaldehyde, mounted in OCT and serially sectioned. Representative sections from the scar region were then stained with the following antibodies: anti-F4/80, anti-MPO (Abcam). Images were acquired using a Zeiss AxioImager and cells were counted using the ‘cell counter’ plugin in ImageJ: at least four fields of view per section were quantified from ≥3 sections per heart. Western blotting Post-MI hearts were lysed in Lamni buffer and proteins resolved on a 2D SDS–PAGE gel. Western blotting was performed using standard methods with antibodies against TNF-α, IL-6, IL-10 (Abcam) and GAPDH (Chemicon). Scanning densitometry was performed and signal quantified using ImageJ. Flow cytometry To measure murine macrophages post MI, hearts isolated post MI were digested into a single-cell suspension using 0.1% collagenase type II (Worthington Biochemical) and cells were stained using a standard protocol with the following antibodies (all from BD Biosciences unless stated otherwise): anti-CD90-APC-Cy7, 53-2.1, anti-B220-PE, RA3-6B2, anti-CD49b-PE, DX5, anti-NK1.1-PE, PK136, anti–Ly-6G-PE, 1A8, anti-CD11b-APC, M1/70, anti-F4/80-biotin, C1:A3-1 (AbD Serotec), anti-CD11c-biotin, HL3, anti-I-A b -biotin, AF6-120.1, anti-Ly-6C-FITC, AL-21, Strep-PE-Cy7 was used to label biotinylated antibodies. Monocytes were identified as CD11b hi (CD90/B220/CD49b/NK1.1/Ly-6G) lo (F4/80/I-A b /CD11c) lo Ly-6C hi/lo . Macrophages/dendritic cells were identified as CD11b hi (CD90.2/B220/CD49b/NK1.1/Ly-6G) lo (F4/80/I-A b /CD11c) hi Ly-6C lo . The sub-population percentage was expressed relative to the total number of cells detected by the cytometer unless otherwise stated. To measure murine peritoneal macrophages, cells were incubated with IFN-γ (10 ng ml −1 ) and Tβ4-SO (100 ng ml −1 ) for 16 h and then isolated on ice for 30 min, followed by centrifugation. Cells were then washed once in PBS and stained using a standard protocol for flow cytometry with the following: anti–Ly-6G-PE, 1A8 (BD Biosciences), anti-CD11b-APC, M1/70 (BD Biosciences), DAPI (Sigma), dihydroethidium (1 μm). For FACS experiments with human cells, cells were isolated as above, washed once in PBS, fixed using 2% paraformaldehyde and stained for flow cytometry with the following antibodies: anti-CD4-PerCP-Cy5.5 (BD Biosciences), anti-CD14-APC (Serotec), anti-CD163-FITC (Santa Cruz Biotechnology), anti-CD206-PE (Immunotec), anti-CD25-PE (Miltenyi Biotech), anti-CD28-FITC (Serotec), anti-CD69-FITC (Serotec) and anti-Ox40-PE (Biolegend). Anti-CD16 AF488 (Biolegend), anti-CD14-APC-cy7 (Biolegend), anti-CD40 PE (Serotech), anti-HLA-DR PerCP-cy5.5 (BD), anti-CD86 Pacific Blue (Biolegend) and anti-CD54 AF647 (Biolegend). Murine and human samples were acquired on a BD LSRII equipped with four lasers (350, 405, 488 and 633 nm) and BD Canto II analyser, respectively, using FACSDiva and FlowJo software. MRI analysis Wild-type C57BL/6J mice treated with Tβ4 or vehicle, were subjected to MRI 7 days after left anterior descending artery ligation. In cases where infarct size was within the range of 15–40%, longitudinal studies were performed at 14 and 28 days post MI. Mice were anaesthetized with isoflurane (4%) and maintained at 37±0.5 °C with oxygen and anaesthetics (1–2% isoflurane), supplied via a nose cone (1 l min −1 ). Cardiorespiratory monitoring and gating were performed using an MR-compatible system (SA Instruments) with needle electrodes inserted into the front limbs and a respiratory pillow placed on the chest. Imaging was performed using a 9.4T VNMRS horizontal bore scanner (Varian) with a shielded gradient system (1,000 mTm−1) using a 39-mm diameter volume coil (Rapid Biomedical GmbH). An electrocardiogram- and respiratory-gated spoiled gradient echo sequence was used to acquire cine cardiac images with the following parameters for standard cine acquisitions: Time to echo (TE), 1.18 ms; time to repetition (TR), 4.5 ms; flip angle, 20°; slice thickness, 1 mm; no slice separation, field of view (FOV), 25.6 × 25.6 mm 2 ; matrix size, 128 × 128; number of signal averages (NSA), 2. Twenty cine-frames were recorded to cover the cardiac cycle. Infarct size was assessed using LGE: 0.6 mmol kg −1 Gd-DTPA was administered i.p. followed by a Look-Locker acquisition with multiple time to inversion (TI) to determine the optimum TI, and by a multi-slice inversion recovery acquisition with flip angle (FA)=90° using the following imaging parameters: TE, 1.58 ms; TR, ~500–600 ms; FA, 90°; slice thickness, 0.5 mm; 0.5 mm slice gap; 7–8 slices; FOV, 25.6 × 25.6 mm 2 ; matrix size, 192 × 192; NSA, 2. A second stack of short-axis images offset by 0.5 mm was acquired to generate a continuous data set. Randomized and anonymized images were analysed using the cardiac analysis software Segment ( http://segment.heiberg.se ). To estimate infarct size, endocardial and epicardial borders were segmented on LGE images automatically with manual adjustments followed by automatic delineation of infarct tissue using a built-in fraction of segment. Infarct size, expressed as percentage of LVM, was calculated as infarct volume/left ventricular volume (from cine data). Comparisons between groups were performed using a repeated measures one-way analysis of variance, using R software25 version 2.8.1. Mouse peritoneal macrophage isolation and assessment of ROS Adult wild-type C57BL/6J mice were humanely euthanized in accordance with A(SP)A 1986, injected i.p. with 5 ml at 4 °C PBS and then agitated to release macrophages from the peritoneal cavity. The PBS containing the cells was re-isolated and the cells centrifuged at 600 g for 10 min and washed once with PBS. Cells were then resuspended in RPMI medium 1640 supplemented with 1% penicillin/streptomycin, 1% glutamine, and 10% heat-inactivated FCS and allowed to adhere to the surface of a 24-well plate for 3 h. Non-adherent (non-macrophage) cells were removed from the well with vigorous washing and macrophages were stimulated with IFN-γ (50 ng ml −1 ), PBS supplemented with 100 ng ml −1 of Tβ4-SO or PBS alone. Peripheral blood cell isolation Ethical approval for the use of peripheral blood from healthy donors was obtained from the Bromley Research Ethics Committee and all subjects provided informed consent. Peripheral blood mononuclear cells were isolated by density-gradient centrifugation (lymphocyte separation media; PAA, Pasching, Austria). Purification of cell subsets was performed by magnetic cell sorting (Miltenyi Biotec) and confirmed by flow cytometry. Monocytes (>90% pure) were isolated by positive selection using anti-CD14 microbeads and T cells also by positive selection using anti-CD4 microbeads (Miltenyi Biotec). Human cell culture Peripheral blood was collected from healthy volunteers, following written informed consent. Ethics approval for this study was given by the Bromley Research Ethics Committee (reference 06/Q0705/20). Mononuclear cells were isolated from PB using Ficoll-Hypaque (LSM 1077; PAA Laboratories) density-gradient centrifugation. Bulk CD4 + T cells (1 × 10 6 per ml) were cultured in 24-well plates in the absence or presence of monocytes in RPMI medium 1640 supplemented with 1% penicillin/streptomycin, 1% glutamine and 10% heat-inactivated FCS (Cambrex, Nottingham, UK) and cultures were stimulated with 100 ng ml −1 anti-CD3 (OKT3; Ortho Biotech, Bridgewater, NJ). In co-culture, 0.5 × 10 6 monocytes were cultured at a 1:1 ratio with CD4 + T cells for 3 days in 24-well plates. Where indicated, cells were also treated with Tβ4 (100 ng ml −1 ), Tβ4-SO (100 ng ml −1 ) or PBS. Quantification of adherence and death of human monocytes Following 3 days in culture, non-adherent and adherent cells were removed separately taking first the media for non-adherent cells and then adding ice-cold PBS before detaching the adherent cells incubated on ice. The number of non-adherent and dead monocytes was then quantified using a trypan blue exclusion assay. ELISA Supernatants were collected and analysed for IFN-γ (R&D Systems) and analysed as per the manufacturer’s instructions. How to cite this article: Evans, M. A. et al . Thymosin β4-sulfoxide attenuates inflammatory cell infiltration and promotes cardiac wound healing. Nat. Commun. 4:2081 doi: 10.1038/ncomms3081 (2013).